Genome-wide microRNA screening reveals that the evolutionary conserved miR-9a regulates body growth by targeting sNPFR1/NPYR MicroRNAs (miRNAs) regulate many physiological processes including body growth. Insulin/IGF signalling is the primary regulator of animal body growth, but the extent to which miRNAs act in insulin-producing cells (IPCs) is unclear. Here we generate a UAS-miRNA library of Drosophila stocks and perform a genetic screen to identify miRNAs whose overexpression in the IPCs inhibits body growth in Drosophila . Through this screen, we identify miR-9a as an evolutionarily conserved regulator of insulin signalling and body growth. IPC-specific miR-9a overexpression reduces insulin signalling and body size. Of the predicted targets of miR-9a , we find that loss of miR-9a enhances the level of sNPFR1. We show via an in vitro binding assay that miR-9a binds to sNPFR1 mRNA in insect cells and to the mammalian orthologue NPY2R in rat insulinoma cells. These findings indicate that the conserved miR-9a regulates body growth by controlling sNPFR1/NPYR -mediated modulation of insulin signalling. Insulin/IGF signalling is a critical pathway regulating body growth from flies to humans [1] . The Drosophila genome contains eight insulin-like peptides (Dilps) whose expression have all been confirmed via in situ hybridization [2] , [3] . Of the seven fly Dilps, Dilp2, 3 , and 5 are expressed in the fly brain in the neurosecretory insulin-producing cells (IPCs). Dilp2 seems to be the most important for proper body growth and longevity [1] , [2] with Dilp2 overexpression in the IPCs enhancing body growth and Dilp2 loss-of-function inhibiting it [1] , [4] . Neuropeptides also play important roles in the physiology and behaviours of animals. In Drosophila , short neuropeptide F (sNPF) regulates body growth by binding to its receptor sNPFR1 in the IPCs and activating ERK-mediated Dilp expression [5] , [6] . As the Dilp peptides are secreted and circulated in the body, they activate the insulin signalling cascade in target tissues resulting in body growth [2] . Thus, sNPF–sNPFR1 signalling modulates Dilp expression, which, in turn, modulates systemic growth, metabolism and lifespan [5] . Like the insulin signalling pathway itself, aspects of this peptidergic insulin control system are evolutionarily conserved. Mammalian neuropeptide Y receptors (NPYRs) show significant homology with sNPFR1 (ref. 7 ) and treatment of rat insulinoma cells with the mammalian sNPF orthologue NPY enhances their expression of insulin [5] . MicroRNAs (miRNAs) are endogenous noncoding RNAs that act as post-transcriptional regulators of gene expression by binding to the 3′-untranslated region (UTR) of target mRNAs. miRNAs exert their effects by suppressing the translation and often inducing the degradation of their target mRNAs. miRNAs play important roles in the regulation of development, stress responses, angiogenesis, oncogenesis and diabetes [8] . Here we report the results of a Drosophila UAS-miRNA library screen that identifies the conserved miR-9a as a regulator of insulin signalling and body growth. Furthermore, we identify Drosophila sNPFR1 and its mammalian orthologue NPY2R as targets of miR-9a in IPCs. Since the insulin and growth phenotypes are rescued by expression of sNPFR1, we propose that the conserved miR-9a/miR-9 regulates body growth by modulating insulin signalling through its conserved sNPFR1/NPY2R target in both Drosophila and mammals. Genome-wide miRNA screen identifies growth regulators To identify miRNAs involved in growth regulation, we generated a library of 131 UAS-miRNA lines covering 144 Drosophila miRNAs ( Supplementary Fig. 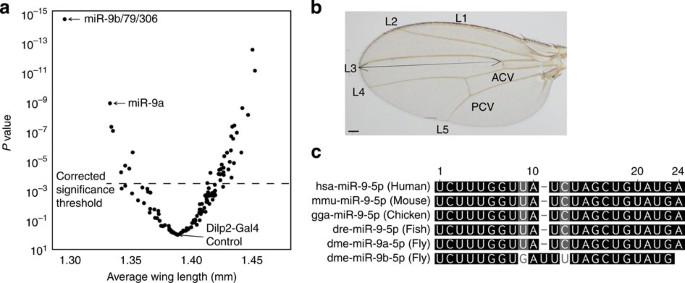Figure 1:miRNAlibrary screen identifies regulators of body growth. (a) A volcano plot of the mean wing lengths of flies whose IPCs overexpress various miRNAs versus their respectivePvalues derived from a one-way analysis of variance followed by pairwiset-tests and a Bonferroni correction for multiple comparisons. All points above the Bonferroni-adjusted significance threshold of 3.79 × 10−4indicated by the dotted line can be considered significant. SeeSupplementary Table 2for a full list of these data points. (b) Wing length was measured from the anterior cross vein (ACV) to the end of the third longitudinal vein (L3) (c) Mature miRNA sequences indicate the degree of conservation in themiR-9family in humans, mice, chickens, zebrafish and fruit flies. Scale bar, 100 μm. 1 and Supplementary Table 1 for details) and crossed them each to the brain IPC driver line Dilp2 - Gal4 (Dilp2>). We then measured progeny wing length from the anterior cross vein (ACV) to the tip of the third longitudinal vein (L3) using the image analysis programme Image J ( Fig. 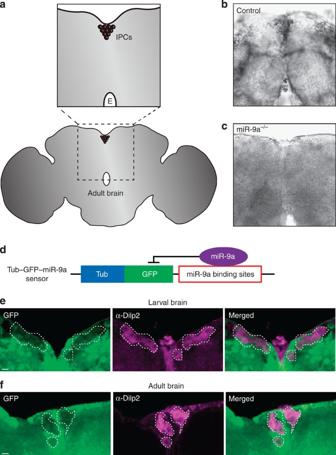Figure 2:miR-9ais expressed in the insulin-producing cells. (a) Adult brain schematics indicate the position of the IPCs in the median neurosecretory cluster in thepars intercerebralis. The ‘E’ indicates the oesophagus. Anin situhybridization with an LNA probe specific to the maturemiR-9asequence stains the IPCs in thew1118control genotype (b), but not inmiR-9aE39/J22null mutant(miR-9a−/−) brains (c). (d) ATubulin–GFP–miR-9asensor schematic. (e,f) TheTubulin–GFP–miR-9asensor shows reduced GFP fluorescence in both the larval (e) and adult (f) IPCs, which are marked by an anti-Dilp2 antibody and with dotted white lines. Scale bar, 10 μm. 1a,b ; Supplementary Table 2 ). The overexpression of many miRNAs in the IPCs alters wing length, both positively and negatively. Figure 1a compares the mean wing length (as measured from the ACV to the tip of L3, Fig. 1b ) induced by the overexpression of various miRNAs to their associated P values. The largest and most significant reductions in wing length are induced by overexpression of miR-9a , miR-9b and miR-79 , which are all members of the conserved miR-9 miRNA family ( Fig. 1c ). The larger reduction in wing length observed for the UAS-miR-9b/79/306 line, which induces overexpression of both miR-9b and miR-79 , is consistent with the fact that both miR-9b and miR-79 have very similar sequences and are likely capable of regulating the same targets. Since UAS-miR-9a significantly reduces wing length via overexpression of a single miRNA, simplifying subsequent analyses, we focused the rest of our efforts on miR-9a . Figure 1: miRNA library screen identifies regulators of body growth. ( a ) A volcano plot of the mean wing lengths of flies whose IPCs overexpress various miRNAs versus their respective P values derived from a one-way analysis of variance followed by pairwise t -tests and a Bonferroni correction for multiple comparisons. All points above the Bonferroni-adjusted significance threshold of 3.79 × 10 −4 indicated by the dotted line can be considered significant. See Supplementary Table 2 for a full list of these data points. ( b ) Wing length was measured from the anterior cross vein (ACV) to the end of the third longitudinal vein (L3) ( c ) Mature miRNA sequences indicate the degree of conservation in the miR-9 family in humans, mice, chickens, zebrafish and fruit flies. Scale bar, 100 μm. Full size image miR-9a is expressed in the insulin-producing cells of brains To investigate the mechanism by which miR-9a alters growth, we used a locked nucleic acid (LNA) probe specific to the mature form of miR-9a in an in situ hybridization experiment. This allowed us to visualize miR-9a expression in larval and adult brains. The IPCs comprise a bundle of bilaterally symmetric neurosecretory cells located dorsally along the midline of the protocerebrum in a region called the pars intercerebralis (PI) ( Fig. 2a ). We observed staining associated with miR-9a probe binding in both the larval ( Supplementary Fig. 2 ) and adult PI regions in a control genotype ( w 1118 ) ( Fig. 2b ; Supplementary Fig. 2b ), but not in homozygous miR-9a −/− null mutant brains stained under identical conditions ( Fig. 2c ; Supplementary Fig. 2c ). Although this staining seems to be widespread, its absence in the miR-9a mutants is consistent with some level of endogenous miR-9a expression in the IPCs of both larvae and adults ( Fig. 2 ; Supplementary Fig. 2 ). To further verify the expression of miR-9a in larval and adult IPCs, we examined Tubulin–GFP–miR-9a sensor lines [9] ( Fig. 2d ) whose ubiquitous expression of GFP is suppressed in miR-9a -expressing cells. The larval and adult IPCs in the Tubulin–GFP–miR-9a sensor flies, here identified by a Dilp2-specific antibody, exhibit less GFP staining than surrounding cells ( Fig. 2e,f ). Thus, both our in situ hybridization and Tubulin–GFP–miR-9a sensor results demonstrate miR-9a expression in both larval and adult IPCs. Figure 2: miR-9a is expressed in the insulin-producing cells. ( a ) Adult brain schematics indicate the position of the IPCs in the median neurosecretory cluster in the pars intercerebralis . The ‘E’ indicates the oesophagus. An in situ hybridization with an LNA probe specific to the mature miR-9a sequence stains the IPCs in the w 1118 control genotype ( b ), but not in miR-9a E39/J22 null mutant ( miR-9a −/− ) brains ( c ). ( d ) A Tubulin–GFP–miR-9a sensor schematic. ( e , f ) The Tubulin–GFP–miR-9a sensor shows reduced GFP fluorescence in both the larval ( e ) and adult ( f ) IPCs, which are marked by an anti-Dilp2 antibody and with dotted white lines. Scale bar, 10 μm. Full size image miR-9a regulates growth and insulin signalling We next increased miR-9a expression in the IPCs using UAS-miR-9a ( Dilp2>miR-9a ) and reduced miR-9a expression in the IPCs using UAS-miR-9a sponge ( Dilp2>miR-9a sponge ). The UAS-miR-9a sponge contains 10 × miR-9a binding sites and tissue specifically reduces miR-9a levels by soaking up endogenous miR-9a molecules [10] . We found miR-9a overexpression in the IPCs ( Dilp2>miR- 9a) reduces body length, wing length and pupal volume, while miR-9a knockdown in the IPCs ( Dilp2>miR-9a sponge ) increases body length, wing length and pupal volume ( Fig. 3a–c ; Supplementary Fig. 3a ). Since insulin/IGF signalling is a major determinant of body growth from flies to human [1] , we tested Dilp levels in these same flies. Although manipulation of miR-9a does not alter larval Dilp5 expression, IPC overexpression of miR-9a ( Dilp2>miR-9a ) reduces larval Dilp2 and Dilp3 mRNA levels, while reduction of miR-9a ( Dilp2>miR-9a sponge ) significantly increases larval Dilp2 mRNA levels ( Fig. 3d–f ). Consistently, IPC overexpression of miR-9a ( Dilp2>miR-9a ) also reduces Dilp2, 3 and 5 mRNA levels, while reduction of miR-9a ( Dilp2>miR-9a sponge ) significantly increases Dilp2 mRNA levels ( Supplementary Fig. 4a,c,e ) in adult heads. Thus, miR-9a in the IPCs seems to regulate body growth via modulation of insulin expression. 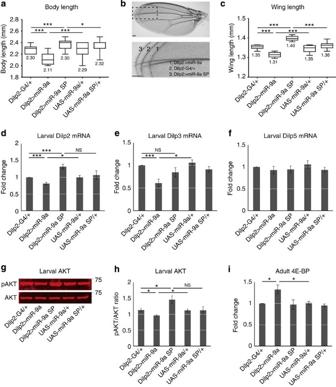Figure 3:miR-9aregulates growth and insulin signalling. (a) When compared with the heterozygousDilp2-Gal4/+,UAS-miR-9a/+andUAS-miR-9a sponge/+controls, overexpression ofmiR-9ain the IPCs (Dilp2>miR-9a) reduces body length, whilemiR-9aknockdown via amiR-9a sponge(Dilp2>miR-9a sponge) increases body length. (b) Superimposed wing images demonstrate the degree to whichmiR-9amodulates wing size. (b,c) Overexpression ofmiR-9areduces wing length, whilemiR-9aknockdown increases wing length. (d–f) IPC-specificmiR-9aoverexpression reduces larval expression ofDilp2 and 3(Dilp2>miR-9a), whilemiR-9aknockdown increases larval expression ofDilp2(Dilp2>miR-9a sponge). Values are normalized to theDilp2-Gal4/+control.Dilp5levels remain unchanged bymiR-9amanipulation. (g,h) Fluorescent western blot visualization of pAKT versus AKT. Larval IPC-specificmiR-9aoverexpression (Dilp2>miR-9a) reduces activated pAKT, whilemiR-9a knockdown(Dilp2>miR-9a sponge) increases activated pAKT. (i) Adult IPC-specific overexpression ofmiR-9aincreases4E-BPlevels compared with theDilp2-Gal4/+andUAS-miR-9a/+controls. Data ind–iare presented as mean±s.e.m. from at least three independent experiments. Statistical significance was assessed by two-tailed Student’st-test; NS, not significant,*P<0.05,***P<0.001. Scale bar, 100 μm. Figure 3: miR-9a regulates growth and insulin signalling. ( a ) When compared with the heterozygous Dilp2-Gal4/+ , UAS-miR-9a/+ and UAS-miR-9a sponge/+ controls, overexpression of miR-9a in the IPCs ( Dilp2>miR-9a ) reduces body length, while miR-9a knockdown via a miR-9a sponge ( Dilp2>miR-9a sponge ) increases body length. ( b ) Superimposed wing images demonstrate the degree to which miR-9a modulates wing size. ( b , c ) Overexpression of miR-9a reduces wing length, while miR-9a knockdown increases wing length. ( d – f ) IPC-specific miR-9a overexpression reduces larval expression of Dilp2 and 3 ( Dilp2>miR-9a ), while miR-9a knockdown increases larval expression of Dilp2 ( Dilp2>miR-9a sponge ). Values are normalized to the Dilp2-Gal4/+ control. Dilp5 levels remain unchanged by miR-9a manipulation. ( g , h ) Fluorescent western blot visualization of pAKT versus AKT. Larval IPC-specific miR-9a overexpression ( Dilp2>miR-9a ) reduces activated pAKT, while miR-9a knockdown ( Dilp2>miR-9a sponge ) increases activated pAKT. ( i ) Adult IPC-specific overexpression of miR-9a increases 4E-BP levels compared with the Dilp2-Gal4/+ and UAS-miR-9a/+ controls. Data in d – i are presented as mean±s.e.m. from at least three independent experiments. Statistical significance was assessed by two-tailed Student’s t -test; NS, not significant, *P <0.05, ***P <0.001. Scale bar, 100 μm. Full size image We next measured AKT phosphorylation and the expression of the dFOXO target gene 4E-BP in an effort to assess insulin signalling in insulin target tissues. When insulin signalling is activated in the target tissues, AKT phosphorylation is increased and 4E-BP expression is reduced because of the reduced nuclear localization of dFOXO. As expected, overexpression of miR-9a in the IPCs ( Dilp2>miR-9a ) reduces the level of pAKT in both larvae ( Fig. 3g,h ) and adults ( Supplementary Fig. 5a ) and increases the level of 4E-BP in adults ( Fig. 3i ). Reduction of miR-9a in the IPCs (Dilp2>miR-9a sponge ) increases the level of pAKT in larvae ( Fig. 3g,h ). In addition, the levels of haemolymph glucose and trehalose rise with miR-9a overexpression and fall with miR-9a knockdown ( Supplementary Fig. 6a ). These results indicate that miR-9a modulates body growth and metabolism by regulating IPC insulin expression and consequently insulin signalling in peripheral target tissues. In further confirmation of our findings, Dilp2 expression in miR-9a −/− null mutant flies is increased like in flies whose IPCs express the miR-9a sponge ( Fig. 4c ). Similar to our findings in Dilp2>miR-9a sponge flies, pAKT levels are increased and 4E-BP levels are decreased in the insulin target tissues of miR-9a −/− null mutants ( Fig. 4f–h ; Supplementary Fig. 5b ). Glucose and trehalose are also reduced in miR-9a −/− null mutant haemolymph as in the Dilp2>miR-9a sponge flies ( Supplementary Fig. 6b ). The body length, wing length and pupal volume of miR-9a −/− null mutants, however, are all reduced ( Fig. 4a,b ; Supplementary Fig. 3b ), in seeming contrast with the results we observed in the Dilp2>miR-9a sponge flies. This suggests that miR-9a in non-IPCs may affect body growth differently than miR-9a in the IPCs. In addition, we show that IPC-specific miR-9a overexpression rescues the Dilp2 expression of the null mutant ( Fig. 4c–e ; Supplementary Fig. 4b,d,f ). 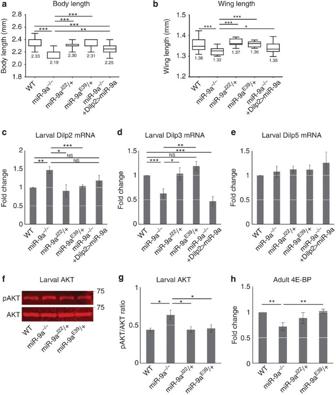Figure 4: IPC-specificmiR-9aoverexpression rescuesDlip2expression of themiR-9anull mutant. (a,b) TransheterozygousmiR-9aE39/J22null mutants show reduced body and wing size compared withWT, miR-9aJ22/+ andmiR-9aE39/+ heterozygous controls, but this growth defect is rescued via IPC-specificmiR-9aoverexpression (miR9a−/−+Dilp2>miR-9a). (c–e)miR-9aE39/J22null mutants have higher larvalDilp2expression and lowerDilp3expression thanWT, miR-9aJ22/+ andmiR-9aE39/+ heterozygous controls.Dilp2expression is restored inmiR-9aE39/J22null mutants by simultaneous IPC-specificmiR-9aoverexpression (miR9a−/−+Dilp2>miR-9a), butDilp3expression is further reduced. (f,g) Larval activated pAKT is elevated inmiR-9aE39/J22null mutants when compared withWT, miR-9aJ22/+ andmiR-9aE39/+ heterozygous controls. (h) Adult4E-BPexpression is reduced in themiR-9aE39/J22null mutants compared withWT, miR-9aJ22/+ andmiR-9aE39/+ heterozygous controls. Data are presented as mean±s.e.m. from at least three independent experiments. Statistical significance was assessed by two-tailed Student’st-test; NS, not significant,*P<0.05,**P<0.01,***P<0.001. Figure 4: IPC-specific miR-9a overexpression rescues Dlip2 expression of the miR-9a null mutant. ( a , b ) Transheterozygous miR-9a E39/J22 null mutants show reduced body and wing size compared with WT, miR-9a J22 /+ and miR-9a E39 /+ heterozygous controls, but this growth defect is rescued via IPC-specific miR-9a overexpression ( miR9a −/− +Dilp2>miR-9a ). ( c – e ) miR-9a E39/J22 null mutants have higher larval Dilp2 expression and lower Dilp3 expression than WT, miR-9a J22 /+ and miR-9a E39 /+ heterozygous controls. Dilp2 expression is restored in miR-9a E39/J22 null mutants by simultaneous IPC-specific miR-9a overexpression ( miR9a −/− +Dilp2>miR-9a ), but Dilp3 expression is further reduced. ( f , g ) Larval activated pAKT is elevated in miR-9a E39/J22 null mutants when compared with WT, miR-9a J22 /+ and miR-9a E39 /+ heterozygous controls. ( h ) Adult 4E-BP expression is reduced in the miR-9a E39/J22 null mutants compared with WT, miR-9a J22 /+ and miR-9a E39 /+ heterozygous controls. Data are presented as mean±s.e.m. from at least three independent experiments. Statistical significance was assessed by two-tailed Student’s t -test; NS, not significant, *P <0.05, **P <0.01, ***P <0.001. Full size image To further support the differential effects of miR-9a in the IPCs and in non-IPCs on body growth, we generated a Dilp2-Gal80 ts line that suppresses Gal4 activity in the IPCs at the 18 °C permissive temperature but not at the 29 °C restrictive temperature. We first verified the function of the Dilp2-Gal80 ts line by confirming that it specifically suppresses in the larval IPCs, the otherwise ubiquitous GFP signal conferred by Tub>GFP ( Fig. 5a ). When miR-9a expression is suppressed outside the IPCs ( Dilp2-G80 ts ; Tub>miR-9a sponge , 18 °C), body length is significantly reduced compared with the Dilp2-G80 ts ; Tub-Gal4 control but Dilp2 expression is unchanged ( Fig. 5b,c ). When miR-9a is suppressed everywhere by shifting the Dilp2-G80 ts ; Tub>miR-9a sponge flies to the restrictive temperature, body length is also reduced and Dilp2 expression is increased like the phenotype we observed in miR-9a −/− null mutant flies (compare Fig. 5b,c with Fig. 4a,c ). These data reveal that miR-9a in the IPCs and in non-IPCs affect body growth differently. 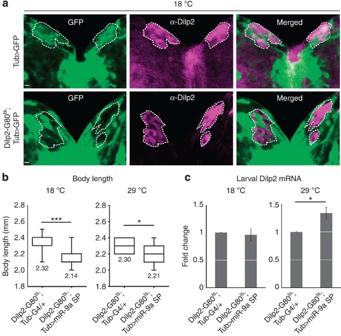Figure 5:miR-9ainside and outside the IPCsdifferentially affects body growth. (a) At the permissive temperature of 18 °C, theDilp2-Gal80tstransgene blocks ubiquitous GFP expression (Tub>GFP)in the larval IPCs, as indicated by anti-Dilp2 staining (magenta). (b,c) Suppression ofmiR-9aexpression outside the IPCs (Dilp2-G80ts; Tub>miR-9a sponge, 18 °C) significantly reduces body length but does not affectDilp2expression. WhenDilp2-Gal80tsis inactivated at 29 °C andmiR-9ais ubiquitously suppressed (Dilp2-G80ts; Tub>miR-9a sponge), body length is less significantly reduced butDilp2expression is increased. Data are presented as mean±s.e.m. from at least three independent experiments. Statistical significance was assessed by two-tailed Student’st-test,*P<0.05,***P<0.001. Scale bar, 10 μm. Figure 5: miR-9a inside and outside the IPCs differentially affects body growth. ( a ) At the permissive temperature of 18 °C, the Dilp2-Gal80 ts transgene blocks ubiquitous GFP expression ( Tub>GFP) in the larval IPCs, as indicated by anti-Dilp2 staining (magenta). ( b , c ) Suppression of miR-9a expression outside the IPCs ( Dilp2-G80 ts ; Tub>miR-9a sponge , 18 °C) significantly reduces body length but does not affect Dilp2 expression. When Dilp2-Gal80 ts is inactivated at 29 °C and miR-9a is ubiquitously suppressed ( Dilp2-G80 ts ; Tub>miR-9a sponge ), body length is less significantly reduced but Dilp2 expression is increased. Data are presented as mean±s.e.m. from at least three independent experiments. Statistical significance was assessed by two-tailed Student’s t -test, *P <0.05, ***P <0.001. Scale bar, 10 μm. Full size image sNPFR1 and its orthologue NPY2R are targets of miR-9a Since the sequence of mature miR-9a is well-conserved from flies to humans ( Fig. 1c ), we reasoned that the miR-9a target responsible for the growth control phenotype may also be conserved. Of the candidate miR-9a targets predicted by Targetscan ( www.targetscan.org ) and miRanda ( www.microRNA.org ), we selected sNPFR1 and its mammalian orthologue NPY2R for further analysis because of their conservation and known regulation of body growth via modulation of insulin expression [5] , [7] . The 3′-UTRs of both sNPFR1 and NPY2R have predicted miR-9a binding sites ( Fig. 6a,d ). We performed a cross-linking immunoprecipitation (CLIP) assay to determine whether miR-9a binds directly to the sNPFR1 and NPY2R 3′-UTRs. In the CLIP technique, miRNA-directed Argonaute-1 (AGO1) binding to a target mRNA followed by ultraviolet cross-linking, immuno-precipitation and subsequent proteinase treatment results in molecules of mRNA cross-linked to short AGO1-derived peptides that interfere with proper reverse transcription to complementary DNA (cDNA). This means 3′-UTR fragment clones of legitimate miRNA targets contain small deletions surrounding the site of AGO1 cross-linking, which is often in or near the miRNA seed sequence crucial for target mRNA pairing [11] , [12] . We performed the CLIP assay on Drosophila S2 and rat INS-1 cells transfected with miR-9a or a scrambled synthetic miRNA . We were able to observe several two to six nucleotide deletions in the miR-9a seed sequence matches of random sNPFR1 and NPY2R 3′-UTR clones from both cell types transfected with miR-9a ( Fig. 6a,d ; Supplementary Table 5 ). This confirms that miR-9a binds to the 3′-UTRs of sNPFR1 and NPY2R . 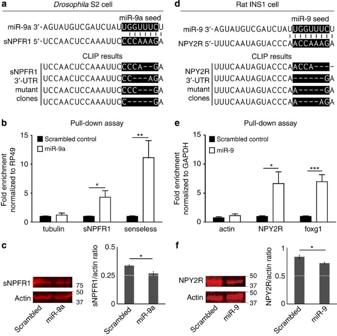Figure 6:miR-9aregulates the insulin modulatorsNPFR1and its mammalian orthologueNPY2R. (a,d; above) Alignment of the maturemiR-9asequence with its predicted target sequences in the 3′-UTRs ofsNPFR1andNPY2R.(a,d; below) MutantsNPFR1andNPY2R3′-UTR clones induced in CLIP assays inDrosophilaS2 and rat INS-1 cells, respectively. (b,e) miRNA–mRNA–RISC pull-down assays inDrosophilaS2 (b) and rat INS-1 (e) cells reveal clear binding ofmiR-9ato both thesNPFR1andNPY2RmRNAs. Transfection ofmiR-9aleads to enrichment ofsNPFR1andNPY2RmRNAs just like known target mRNAssenselessandfoxg1when normalized torp49andGAPDHlevels. Transfection with a scrambled version ofmiR-9a(Supplementary Table 3) causes no such enrichment. (c,f) Transfection of a syntheticmiR-9aduplex reduces the level of sNPFR1 protein produced by S2 cells (c) and the level of NPY2R protein produced by INS-1 cells (f) when compared with levels produced on transfection with a scrambledmiR-9a(Supplementary Table 3). Data inb,cande,fare presented as mean±s.e.m. from at least three independent experiments. Statistical significance was assessed by two-tailed Student’st-test,*P<0.05,**P<0.01,***P<0.001. Figure 6: miR-9a regulates the insulin modulator sNPFR1 and its mammalian orthologue NPY2R . ( a , d ; above) Alignment of the mature miR-9a sequence with its predicted target sequences in the 3′-UTRs of sNPFR1 and NPY2R. ( a , d ; below) Mutant sNPFR1 and NPY2R 3′-UTR clones induced in CLIP assays in Drosophila S2 and rat INS-1 cells, respectively. ( b , e ) miRNA–mRNA–RISC pull-down assays in Drosophila S2 ( b ) and rat INS-1 ( e ) cells reveal clear binding of miR-9a to both the sNPFR1 and NPY2R mRNAs. Transfection of miR-9a leads to enrichment of sNPFR1 and NPY2R mRNAs just like known target mRNAs senseless and foxg1 when normalized to rp49 and GAPDH levels. Transfection with a scrambled version of miR-9a ( Supplementary Table 3 ) causes no such enrichment. ( c , f ) Transfection of a synthetic miR-9a duplex reduces the level of sNPFR1 protein produced by S2 cells ( c ) and the level of NPY2R protein produced by INS-1 cells ( f ) when compared with levels produced on transfection with a scrambled miR-9a ( Supplementary Table 3 ). Data in b , c and e , f are presented as mean±s.e.m. from at least three independent experiments. Statistical significance was assessed by two-tailed Student’s t -test, *P <0.05, **P <0.01, ***P <0.001. Full size image Next, we performed a miRNA–mRNA pull-down assay for further confirmation of miR-9a binding to the sNPFR1 and NPY2R mRNAs. After transfection with either biotinylated miR-9a or a scrambled miRNA, we isolated the biotin–miRNA–RISC–mRNA complex with streptavidin beads. Similar to the known miR-9a/miR-9 targets senseless [13] and Foxg1 (ref. 14 ), we found that miR-9a binds to and enriches sNPFR1 mRNA over RP49 control RNA in Drosophila S2 cells and NPY2R mRNA over GAPDH control RNA in rat insulinoma INS-1 cells ( Fig. 6b,e ). Consequently, miR-9a transfection reduces sNPFR1 and NPY2R protein levels compared with an actin control in both Drosophila S2 and rat insulinoma cells, respectively ( Fig. 6c,f ). In addition, miR-9a −/− null mutant flies produce significantly more sNPFR1 protein than the wild-type control strain ( Supplementary Fig. 7 ). These results support the hypothesis that the sNPFR1 and NPY2R mRNAs are legitimate targets of miR-9a/miR-9 . To further support our hypothesis that miR-9a inhibits growth and suppresses insulin signalling via its target sNPFR1 , we simultaneously overexpressed both miR-9a and sNPFR1 in the Drosophila IPCs. Indeed, overexpression of sNPFR1 rescues the reduced body and wing length phenotypes of Dilp2>miR-9a flies ( Fig. 7a,b ). Similarly, sNPFR1 overexpression also restores Dilp2 and 3 expression levels ( Fig. 7c–e ). We next asked whether reduced sNPFR1 dosage ( sNPFR1 minos−/+ heterozygote) can restore body length and Dilp2 expression in the background of miR-9a knockdown via miR-9a sponge . The sNPFR1 heterozygote restores body length significantly in the miR-9a sponge ( Dilp2>miR-9a sponge+sNPFR1 minos−/+ ) and slightly in the miR-9a −/− null mutants ( miR-9a −/− +sNPFR1 minos−/+ ) ( Fig. 8a,c ). The sNPFR1 heterozygote also restores Dilp2 expression in the miR-9a sponge and miR-9a −/− null mutant backgrounds ( Dilp2>miR-9a sponge+sNPFR1 minos−/+ or miR-9a −/− +sNPFR1 minos−/+ ) ( Fig. 8b,d ). Finally, we further characterized the wing growth phenotype caused by miR-9a manipulation by measuring both cell size and cell number. Compared with the control ( Dilp2-Gal4/+ ), overexpression of miR-9a in the IPCs ( Dilp2>miR-9a) reduces both wing cell size and number, while knockdown of miR-9a ( Dilp2>miR-9a sponge ) increases wing cell size and number. As expected, the changes in wing cell size and number induced by miR-9a overexpression in the IPCs are rescued by simultaneous overexpression of sNPFR1 ( Dilp2>miR-9a+sNPFR1 ) ( Fig. 7f,g ). These results confirm that miR-9a in IPCs regulates insulin signalling and body growth via its target sNPFR1 ( Fig. 9 ). 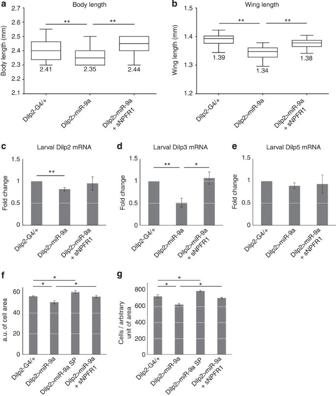Figure 7: SimultaneoussNPFR1overexpression rescues the phenotypes induced bymiR-9aoverexpression. (a,b) Boxplots indicating that the reduced body and wing length phenotypes induced by IPC-specificmiR-9aoverexpression (Dilp2>miR-9a) are rescued by simultaneous overexpression of themiR-9atargetsNPFR1(Dilp2>miR-9a+sNPFR1). (c–e) The reduction ofDilp2and3observed inDilp2>miR-9aflies is rescued inDilp2>miR-9a+sNPFR1flies. (f) The wing growth defect induced by IPC-specificmiR-9aoverexpression (Dilp2>miR-9a) stems from a reduction in both wing cell size and number. This defect can be rescued by simultaneoussNPFR1overexpression (Dilp2>miR-9a+sNPFR1). (g) The increase in wing size observed in theDilp2>miR-9a spongeflies stems from an increase in both cell size and number. Data inc–gare presented as mean±s.e.m. from at least three independent experiments. Statistical significance was assessed by two-tailed Student’st-test,*P<0.05,**P<0.01. Figure 7: Simultaneous sNPFR1 overexpression rescues the phenotypes induced by miR-9a overexpression. ( a , b ) Boxplots indicating that the reduced body and wing length phenotypes induced by IPC-specific miR-9a overexpression ( Dilp2>miR-9a ) are rescued by simultaneous overexpression of the miR-9a target sNPFR1 ( Dilp2>miR-9a+sNPFR1) . ( c – e ) The reduction of Dilp2 and 3 observed in Dilp2>miR-9a flies is rescued in Dilp2>miR-9a+sNPFR1 flies. ( f ) The wing growth defect induced by IPC-specific miR-9a overexpression ( Dilp2>miR-9a ) stems from a reduction in both wing cell size and number. This defect can be rescued by simultaneous sNPFR1 overexpression ( Dilp2>miR-9a+sNPFR1 ). ( g ) The increase in wing size observed in the Dilp2>miR-9a sponge flies stems from an increase in both cell size and number. Data in c – g are presented as mean±s.e.m. from at least three independent experiments. Statistical significance was assessed by two-tailed Student’s t -test, *P <0.05, **P <0.01. 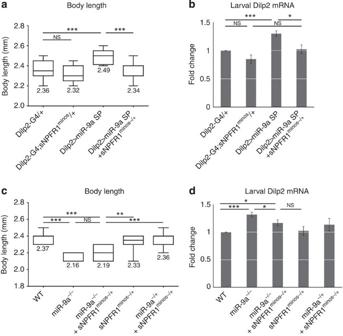Figure 8:sNPFR1heterozygous rescues the body length andDilp2expression by IPC-specific knockdown ofmiR-9a. (a,b) Addition ofsNPFR1minos−/+heterozygosity rescues the body length andDilp2expression phenotype caused bymiR-9aknockdown in the IPCs (Dilp2>miR-9a sponge+sNPFR1minos−/+). Compare with theDilp2>miR-9a sponge, Dilp2-Gal4/+andDilp2-Gal4; sNPFR1minos−/+controls. (c,d)sNPFR1minos−/+heterozygosity also rescues body length andDilp2expression in themiR-9aE39/J22null mutants background (miR9a−/−+sNPFR1minos−/+) compared withmiR-9aE39/J22null mutants.WT, sNPFR1minos−/+andmiR9a−/++sNPFR1minos−/+are the controls. Data are presented as mean±s.e.m. from at least three independent experiments. Statistical significance was assessed by two-tailed Student’st-test, NS, not significant,*P<0.05,**P<0.01,***P<0.001. Full size image Figure 8: sNPFR1 heterozygous rescues the body length and Dilp2 expression by IPC-specific knockdown of miR-9a . ( a , b ) Addition of sNPFR1 minos−/+ heterozygosity rescues the body length and Dilp2 expression phenotype caused by miR-9a knockdown in the IPCs ( Dilp2>miR-9a sponge+sNPFR1 minos−/+ ). Compare with the Dilp2>miR-9a sponge, Dilp2-Gal4/+ and Dilp2-Gal4; sNPFR1 minos−/+ controls. ( c , d ) sNPFR1 minos−/+ heterozygosity also rescues body length and Dilp2 expression in the miR-9a E39/J22 null mutants background ( miR9a −/− +sNPFR1 minos−/+ ) compared with miR-9a E39/J22 null mutants. WT, sNPFR1 minos−/+ and miR9a −/+ +sNPFR1 minos−/+ are the controls. Data are presented as mean±s.e.m. from at least three independent experiments. Statistical significance was assessed by two-tailed Student’s t -test, NS, not significant, *P <0.05, **P <0.01, ***P <0.001. 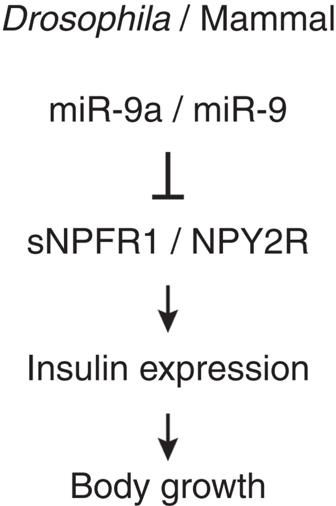Figure 9: A model summarizing the results of this study. . Full size image Figure 9: A model summarizing the results of this study. . Full size image We have uncovered a novel function for miR-9a in the regulation of insulin signalling and body growth through its target sNPFR1 in the Drosophila brain IPCs. In a miRNA overexpression screen using the IPC driver Dilp2-Gal4 , we found that miR-9a and the closely related miR-9b dramatically reduce wing size ( Fig. 1 ). We were able to verify that miR-9a is endogenously expressed in the larval and adult IPCs via LNA in situ hybridization against the mature miRNA and via miR-9a sensor lines ( Fig. 2 ; Supplementary Fig. 2 ). IPC-specific overexpression of miR-9a also reduces body size, while knockdown of miR-9a via expression of a miR-9a sponge increases body size. This effect is likely caused by modulation of insulin expression, as miR-9a overexpression reduces Dilp2 levels, while miR-9a knockdown enhances Dilp2 levels ( Fig. 3 ). Contrary to expectations, we found that while sponge-mediated knockdown of miR-9a in the IPCs increases body size, miR-9a −/− null mutants and flies in which miR-9a is suppressed in non-IPCs show reduced body size. In other words, loss of miR-9a in the IPCs alone increases growth while ubiquitous or non-IPC loss of miR-9a reduces growth ( Figs 3a , 4a and 5b ). We found, however, that the level of Dilp2 mRNA is increased in both Dilp2>miR-9a sponge and miR-9a −/− null mutant flies and the level of the downstream signalling protein pAKT is significantly increased in the miR-9a mutants ( Figs 3d,g and 4c,f ). This activation of insulin signalling in both the miR-9a sponge flies and the miR-9a −/− null mutants suggests that miR-9a has positive effects on growth in non-IPCs that are able to mask its negative effect on growth in the IPCs. In the IPCs, miR-9a is likely mediating its effects by targeting the known positive regulator of insulin expression sNPFR1 as miR-9a −/− null mutants express elevated levels of sNPFR1 ( Supplementary Fig. 7 ). Mammals have multiple NPY receptors, but sNPFR1 is strongly similar to NPY2R (ref. 7 ). The germ-line deletion of NPY2R reduces mouse body weight and adiposity [15] and the sNPFR1 dominant negative mutation reduces fly body growth through ERK [5] . Although the IPCs of invertebrates are localized in the brain and the IPCs of mammals are in the pancreas, the functional similarities of the two systems are clear. sNPF overexpression in flies causes hyperinsulinemia and enhances body growth [5] , while NPY overexpression in mammals causes hyperinsulinemia, hyperphagia and obesity [16] . In mice, a triple knockout of NPY1R, NPY2R and NPY4R prevents the hyperinsulinemia associated with NPY overexpression, indicating that NPY signalling through the NPY receptors modulates insulin secretion [17] . Here we show that both fly sNPFR1 and mammalian NPY2R are targets of miR-9a/miR-9 by demonstrating direct binding of miR-9a/miR-9 to the sNPFR1 and NPY2R 3′-UTRs using an in vitro binding assay and a CLIP assay ( Fig. 6 ). Our results suggest an evolutionarily conserved relationship between the miR-9 family and the sNPF/NPY receptors ( Fig. 9 ). miR-9 in mammals is expressed in both the brain and the pancreatic beta cells where it has been shown to regulate glucose levels via its targets onecut2 and sirt1 (refs 18 , 19 ). In addition to its effects in the brain on pancreatic insulin secretion, NPY is also released by the autonomic nervous system into the pancreas where it directly modulates insulin and glucagon secretion [20] . It will thus be interesting to see if the relationship we have uncovered between the miR-9 , NPY, insulin signalling and body growth extends to in vivo mammalian models despite the differences in anatomical location and embryonic origin of the IPCs. Drosophila culture and stocks All flies were maintained at 25 °C on standard cornmeal, yeast, sugar, agar medium. Wild-type Oregon R, w 1118 and sNPFR1 minos were obtained from the Bloomington Stock Center (Bloomington, USA). Dilp2-Gal4 was provided by E. Rulifson (University of California San Francisco, USA), and miR-9a J22 and miR-9a E39 mutants were provided by F.B. Gao (University of Massachusetts Medical School, USA). miR-9a sponges were provided by D. Van Vactor (Havard medical school, USA). Tubulin–GFP–miR-9a sensor was provided by E. Lai (Sloan-Kettering Institute, USA). The UAS-sNPFR1 transgenic fly was generated by the p-element-mediated germline transformation method with the pUAS–sNPFR1 construct containing the full length of sNPFR1 cDNA in the pUAS vector [5] . To generate the Dilp2-Gal80 ts line, we amplified the Dilp2 promoter ( Supplementary Table 4 for primer sequences) via PCR and inserted it into pBPGAL80Uw-6 (a gift from Y.-J.K.). We then microinjected the resulting construct for site-specific insertion on chromosome 2L (PBac{y+-attP-3B}VK00037 embryos) using standard methods. UAS-miRNA library construction We obtained 45 previously published UAS-DsRed-pre-miRNA constructs from the Drosophila RNAi Screening Center [21] . Using overlapping oligos, we modified these vectors by adding minimal attB sites into the Mlul site to make them suitable for site-specific insertion into the fly genome. To produce the rest of the stocks, we modified an attB-containing SST13 UAS vector [22] , which makes use of the split-white system to reduce time spent on off-target insertions [23] . We inserted additional restriction sites between the KpnI and XbaI sites of the SST13 polylinker using overlapping oligos (5′- CTAGAGCGAGCTCAAGGCCACTAGGGCCGGGATCGATATGGTAC -3′ and 5′- CATATCGATCCCGGCCCTAGTGGCCTTGAGCTCGCT -3′). Inspired by the design of the Silver et al. [21] UAS-miRNA vectors, we also inserted the DsRed coding sequence downstream of a 5 × UAS sequence and renamed this vector pSS-DsRed . Next, we amplified putative pri-miRNA sequences consisting of roughly 400–500 bp surrounding each mature miRNA sequence and inserted them into pSS-DsRed . We validated all the UAS-miRNA vectors with restriction digests and sequencing. See Supplementary Table 1 for a summary of these UAS-miRNA constructs and the primers used to make them. All of our UAS-miRNA constructs were inserted into a specific attP site on the second (VIE-72a, a gift from B. Dickson) or third chromosome (VIE-49b, a gift from B. Dickson) using the ФC31 integrase system and standard transgenesis techniques. miRNA in situ hybridization We performed the miRNA in situ hybridizations on larval and adult Drosophila brains essentially by the standard technique [24] with minor modifications as follows: We fixed the brains for 1 h at room temperature and used methanol for washing instead of ethanol. We did not use any Proteinase K treatment, nor did we do any secondary fixation. We used a DIG-labelled miR-9a-specific LNA probe purchased from Exiqon (#88078-15) at 50 nM for larval brains and 250 nM for adult brains. We performed the hybridization reaction and subsequent washings at 60 °C for larval brains and 65 °C for adult brains. We visualized binding of the LNA probe with an anti-DIG antibody coupled to alkaline phosphatase, developing the larval brains for 80 min and the adult brains for 2 days. The elevated concentration and development time required for the adult in situ may indicate either lower expression or some degree of probe degradation, but the staining was clearly specific as the miR-9a null mutant brains stained at the same time and under the same conditions were blank. Cell culture and transfection We purchased Drosophila S2 cells from the Drosophila Genomics Resource Center (DGRC, the Indiana University) and maintained them at 26 °C in Schneider media supplemented with 10% bovine calf serum. We cultured rat insulinoma INS-1 cells in 5% CO 2 at 37 °C in RPMI 1640 media containing 2 mM L-glutamine supplemented with 10% foetal bovine serum, 5.6 mM glucose, 10 mM HEPES, 1 mM sodium pyruvate, 50 μM 2-mercaptoethanol, 100 IU ml −1 penicillin and 100 μM streptomycin. We transfected the cells with either synthetic scrambled miR-9a or miR-9a duplex (Bioneer, Korea) (final concentration 80 μM) using Xtremegene HP (Roche, USA). The scrambled miR-9a and miR-9a duplex sequences used in the transfection are listed in Supplementary Table 3 . CLIP assay and the miRNA–mRNA pull-down assay We performed the CLIP assay [11] , [25] with the following modifications: 24 h post transfection, we irradiated the cells with 150 mJ cm −2 at 254 nm using a CL-100s UV Cross-linker. We then harvested the cells, added lysis buffer (Cell Signaling, USA) and treated them with a low dose of RNase A (100 ng ml −1 ) for partial RNA digestion. We then used Protein A Dynabeads (Invitrogen, USA) and 2 μg AGO-1-specific antibody for the immuno-precipitation. The immunoprecipitate was treated with 20 μg ml −1 proteinase K for 10 min at 37 °C. We then extracted the RNA using the easy-BLUE kit (iNTRON, Korea) and synthesized cDNAs using the SuperScript III First-Strand Synthesis System (Invitrogen). To determine whether miR-9a directly binds to sNPFR1 and NPY2R mRNA, we designed primers to amplify fragments of their 3′-UTRs that include the predicted miR-9a seed sequence matches ( Supplementary Table 4 ). We used standard PCR and the Zero Blunt TOPO PCR Cloning Kit (Invitrogen) to obtain and then sequence several clones for each condition ( Supplementary Table 5 ). We performed the biotin–RNA pull-down assay [26] with the following modifications: The cells were harvested after transfection for 24 h and lysed in lysis buffer (Cell Signaling) containing 20 × protease inhibitor (Roche) and 60 U RNaseOUT (Invitrogen). We used streptavidin agarose beads (GE Healthcare, UK) for the immuno-precipitation. We extracted the RNA using the easy-BLUE kit and synthesized cDNAs using the SuperScript III First-Strand Synthesis System. We then performed quantitative real-time PCR using primers ( Supplementary Tables 3 and 4 ) specific to fragments of the 3′-UTRs of sNPFR1 and NPY2R that contain the miR-9a seed match. We used senseless and foxg1 as positive controls and actin and tubulin as negative controls. Quantitative RT–PCR analysis We collected heads or bodies from 15 adult flies and isolated total RNA with the easy-BLUE reagent. After treating the RNA samples with RNase-free DNase I (TAKARA, Japan), we synthesized cDNA using the SuperScript III First-Strand Synthesis System. We then performed quantitative reverse transcription–PCR (RT–PCR) analysis with the StepOnePlus Sequence Detection System (Applied Bio Systems, USA) using the SYBR Green PCR Core reagents (Applied Bio Systems). We performed each experiment at least three times and used the comparative cycle threshold to present a fold change for each specific mRNA after normalizing to rp49 levels. The primers we used in our qPCR analyses are listed in Supplementary Table 3 . Fluorescent western blots We isolated total protein from the bodies of adult flies or larvae and from Drosophila S2 cells or rat INS-1 cells with the PROPREP protein extraction buffer (iNtRON) or RIPA buffer (Cell Signaling). We subjected 30 μg of the fly proteins and 80 μg of the cell line proteins to SDS–PAGE and transferred them to low fluorescence PVDF membrane (Thermoscientific, USA). We blocked the membranes for 60 min in TBS buffer containing 5% BSA and incubated them overnight at 4 °C with primary antibodies. After incubation in the dark with fluorophore-tagged secondary antibodies and subsequent washes, we digitized images of the membranes using the Amersham Imager 600 (Amersham Biosciences, USA). We then quantified target protein versus their internal loading control band intensities with the Tina2.0 software (UK). We used the following primary antibodies: anti-phospho-Akt (1:1,000, Cell Signaling), anti-Akt (1:1,000, Cell Signaling), anti-NPY2R (1:1,000, Santa Cruz, USA), anti-β-actin for Drosophila (1:1,000, Developmental Studies Hybridoma Bank, DSHB, USA) and anti-β-actin for mammals (1:1,000, Santa Cruz). We used the following secondary antibodies: Goat anti-rat IgG, Dylight488 (1:1,000, Pierce, USA), Goat anti-mouse IgG, DyLight488 (1:1,000, Thermoscientific), Goat anti-rabbit IgG, DyLight488 (1:1,000, Thermoscientific) and Alexa fluor 680 donkey anti-rabbit IgG (1:500, Life technologies, USA) ( Supplementary Fig. 8 ). Measurement of body length and wing length To avoid artifacts caused by vial over-crowding, we maintained population densities of 50 embryos per vial in standard fly media. Using the Image J analysis package and a microruler, we measured the body length of adult males 3–5 days post eclosion from the anterior end of the head to the posterior end of the abdomen. We measured wing length from the ACV to the end of third longitudinal vein (L3). Measurement of cell size and cell number To quantify relative cell size and cell number, wings were digitally photographed at × 200 magnification. Image J analysis software was used to measure relative pixel areas of wings, using wing vein landmarks to retain fair morphological comparisons. Adobe Photoshop software was used to measure a 100 × 100 pixel area of the L4–L5 inter-vein region. We counted epidermal hairs within this same pixel area to measure relative pixel area per cell or cell size. To calculate relative cell number, the wing pixel area was multiplied by the relative pixel area per cell. Data were collected for males only. Measurement of the haemolymph glucose and trehalose levels We collected 3–5 days–old-adult flies to measure glucose and trehalose levels in haemolymph. To collect the haemolymph, the flies were punched in the thorax and then transferred to 0.5 ml tube placing in a 1.5 ml collection tube. The tubes were then centrifuged at 5,000 r.p.m. for 5 min. About 1 μl of haemolymph was added to 30 μl of 1 × trehalose solution (Sigma, USA) and incubated for 16–18 h at 37 °C. Next, we added Glucose assay (GO) reagent (Sigma) and incubated at 37 °C for 30 min. The reaction was stopped by the addition of 12 N H 2 SO 4 . Total haemolymph glucose concentration (from trehalose and glucose) was measured using microplate reader (BioTek, USA) at 540 nm. Standard curves were generated by D-(+)-glucose solution (Sigma) for every experimental trial. A linear regression of concentration samples over the standard range was used to find actual concentration from haemolymph samples. Statistics Boxplots in this study follow the standard style except that the whiskers represent minimum to maximum. Regarding the bar charts, unless otherwise noted, we present the mean±s.e.m. and make comparisons between groups using the Student’s t -test considering P <0.05 as statistically significant. For the multiple comparisons made in Fig. 1a , we performed a one-way analysis of variance followed by pairwise t -tests using the Bonferroni method to adjust the P value threshold for significance. How to cite this article: Suh, Y. S. et al. Genome-wide microRNA screening reveals that the evolutionary conserved miR-9a regulates body growth by targeting sNPFR1/NPYR. Nat. Commun. 6:7693 doi: 10.1038/ncomms8693 (2015).